Topoisomerase IIα promotes activation of RNA polymerase I transcription by facilitating pre-initiation complex formation Type II DNA topoisomerases catalyse DNA double-strand cleavage, passage and re-ligation to effect topological changes. There is considerable interest in elucidating topoisomerase II roles, particularly as these proteins are targets for anti-cancer drugs. Here we uncover a role for topoisomerase IIα in RNA polymerase I-directed ribosomal RNA gene transcription, which drives cell growth and proliferation and is upregulated in cancer cells. Our data suggest that topoisomerase IIα is a component of the initiation-competent RNA polymerase Iβ complex and interacts directly with RNA polymerase I-associated transcription factor RRN3, which targets the polymerase to promoter-bound SL1 in pre-initiation complex formation. In cells, activation of rDNA transcription is reduced by inhibition or depletion of topoisomerase II, and this is accompanied by reduced transient double-strand DNA cleavage in the rDNA-promoter region and reduced pre-initiation complex formation. We propose that topoisomerase IIα functions in RNA polymerase I transcription to produce topological changes at the rDNA promoter that facilitate efficient de novo pre-initiation complex formation. Topoisomerases cleave DNA to elicit topological changes, facilitating DNA-processing events in cells, including transcription [1] , [2] , [3] . The type II topoisomerases (Top2) relax supercoiled DNA by a double-strand DNA passage reaction. There is much interest in understanding the cellular roles of the Top2 enzymes, the mechanisms and sites of action and the processes involved in recruitment to these sites, particularly as these proteins are targets for clinically important anti-cancer drugs [4] , [5] , [6] . In transcription, Top2 activity has been implicated in resolving supercoiling associated with elongation by RNA polymerases [7] , [8] , [9] , [10] , [11] , [12] . In RNA polymerase I (Pol I) transcription, in yeast, Top2 cleavage resolves the positive supercoiling ahead of the elongating polymerase, whereas Top1 resolves negative torsion behind the polymerase [7] and, in mammalian cells, Top1 has been shown to have an important role in Pol I transcription elongation [13] , [14] , [15] . Mammalian cells have two isoforms of Top2, α and β, with similar enzymatic activities and 68% overall sequence identity, but Top2α and β differ markedly in their C-terminal domains (CTDs), which appear to determine isoform-specific functions. Top2α, specifically, is essential for chromatid segregation and decatenation G2-checkpoint function [16] , [17] , for instance, whereas, Top2β is involved in the repair of DNA cross-links and the transcriptional induction of a subset of hormone- and developmentally regulated genes in Pol II transcription [18] , [19] , [20] , [21] , [22] . To our knowledge, a Top2α-specific role in transcription has not yet been described. Intriguingly, our proteomic analyses of Pol I complexes had revealed, previously, the specific co-purification of Top2α with the initiation-competent Pol Iβ complex [23] . Pol I transcription produces the major ribosomal RNA (rRNA) constituents of the protein-synthesis machinery, driving cell growth and proliferation and, thereby, influencing cell fate [24] , [25] . Upregulation of Pol I transcription is linked to the unrestrained growth and proliferation characteristic of cancer cells [26] , [27] . Here we present evidence for a role for Top2α in the early stages of the Pol I transcription cycle. We demonstrate that Top2α is a component of Pol Iβ and can bind to the RRN3 component of Pol Iβ, which bridges the interaction between Pol I and basal transcription factor SL1 at the rRNA gene promoter [28] , [29] , [30] . We found that drug-induced inhibition of Top2 activity did not prevent elongation of rRNA transcripts. Our data suggest a novel and specific role for Top2α activity in facilitating de novo pre-initiation complex (PIC) formation in rRNA gene transcription. Top2 inhibitors produced a defect in activation of Pol I transcription, independently of the DNA-damage response pathways, suggesting that drugs designed to target Top2α in Pol I transcription could be useful non-genotoxic agents in the treatment of cancer. Active Top2α is a component of initiation-competent Pol Iβ Pol I transcribes the rRNA gene repeats to produce the 47S pre-rRNA transcript that is processed into the 18S, 5.8S and 28S rRNAs [24] , [25] , [28] , [31] . Two functionally distinct forms of Pol I complex can be extracted from the nucleus of human cells. The Pol Iα complex, the most abundant form of Pol I in nuclear extracts, is catalytically active but does not support promoter-specific initiation at an rRNA gene promoter. The Pol Iβ complex accounts for ~10% of Pol I activity and is competent for promoter-specific transcription initiation. Pol Iβ is defined by the association of its Pol I core subunits with growth-regulated transcription initiation factor RRN3, which bridges the interaction between basal transcription factor SL1 and Pol I in formation of functional PICs at the rRNA gene promoter [24] , [25] , [28] . We have previously reported that Top2α co-fractionates with the Pol Iβ promoter-specific transcription activity and is the major substrate for Pol Iβ-associated CK2 in the Pol Iβ complex [23] . We demonstrate that Pol Iβ has an associated decatenation activity that is ATP-dependent and sensitive to non-hydrolysable ATP and Top2 inhibitor etoposide ( Fig. 1a ). The decatenation activity and Top2α protein co-purify with the RRN3 component of Pol Iβ ( Supplementary Fig. S1a ). These data suggest that catalytically active Top2α is associated with the initiation-competent Pol Iβ complex. 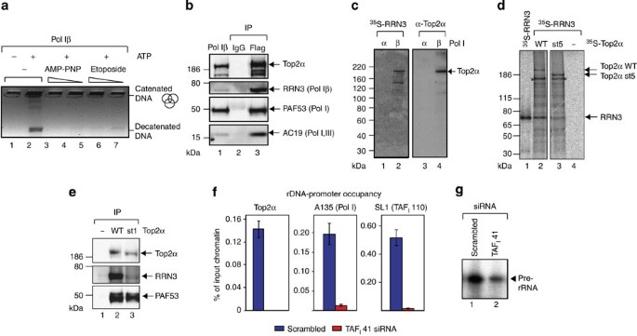Figure 1: Top2α is a component of initiation-competent Pol Iβ and interacts directly with RRN3 and occupies the rDNA promoter. (a) Pol Iβ-associated decatenation activity is ATP-dependent and sensitive to non-hydrolysable ATP and Top2 inhibitor. Pol Iβ peak fractions were incubated +/− ATP, AMP-PNP and etoposide in a kinetoplast DNA decatenation assay. (b) Top2α co-immunoprecipitates with Pol Iβ. Pol I was immunoprecipitated from nuclear extracts of HeLa cells expressing Flag-CAST (Pol I), using Flag-antibodies, and then immunoblotted for Top2α, Pol Iβ subunit RRN3 and Pol I subunits PAF53 and AC19. Purified Pol Iβ (lane 1); IgG immunoprecipitate (lane 2). (c) RRN3 interacts with Top2α of Pol Iβ in far-western analysis. Pol Iα and Iβ were probed with35S-Flag-RRN3 and Top2α-antibodies. (d) Top2α C-terminus is important for RRN3 interaction.In vitro-translated and Flag-immunopurified35S-Flag-RRN3 was incubated within vitro-translated35S-GFP-Top2α WT and C-terminal-truncated (st5; 180 amino-acid deletion) proteins on GFP-antibody beads. Input RRN3 (1%, lane 1); RRN3 with GFP-antibody beads (lane 4); *contaminating translation product. (e) Efficient co-IP of Top2α with Pol Iβ requires its C-terminal 42 amino acids. Top2α was immunoprecipitated from HTETOP cells depleted for endogenous Top2α and stably expressing GFP-Top2α-WT and C-terminal-truncated (st1, 42 amino-acid deletion) proteins, using GFP antibodies. IgG control (lane 1). Immunoprecipitates were immunoblotted using antibodies for Top2α, PAF53 and RRN3. Representative immunoblot is shown. Quantitation and normalization of the RRN3 and PAF53 immunoblot signals to those of Top2α-WT and -st1, in three independent experiments, revealed that C-terminal 42 amino-acid truncation of Top2α reduced RRN3 and PAF53 signals ~sixfold and ~twofold, respectively. (f) Top2α occupancy of the rDNA promoter is reduced in TAFI41-depleted cells with decreased rRNA transcription. HEK293 cells were transfected with scrambled or SL1 subunit TAFI41 (TAF1D) small interfering RNAs (siRNAs). rDNA-promoter occupancy by Top2α, Pol I subunit A135 and SL1 subunit TAFI110 (TAF1C) in these cells was analysed by ChIP using Top2α, A135 and TAFI110 antibodies; data in bar graphs are from three independent ChIP experiments, normalized to control IgG samples; s.d. is shown. (g) Control forfshowing pre-rRNA levels from cells transfected with scrambled siRNA (lane 1) or TAFI41 siRNA (lane 2) as analysed by S1 nuclease protection. Figure 1: Top2α is a component of initiation-competent Pol Iβ and interacts directly with RRN3 and occupies the rDNA promoter. ( a ) Pol Iβ-associated decatenation activity is ATP-dependent and sensitive to non-hydrolysable ATP and Top2 inhibitor. Pol Iβ peak fractions were incubated +/− ATP, AMP-PNP and etoposide in a kinetoplast DNA decatenation assay. ( b ) Top2α co-immunoprecipitates with Pol Iβ. Pol I was immunoprecipitated from nuclear extracts of HeLa cells expressing Flag-CAST (Pol I), using Flag-antibodies, and then immunoblotted for Top2α, Pol Iβ subunit RRN3 and Pol I subunits PAF53 and AC19. Purified Pol Iβ (lane 1); IgG immunoprecipitate (lane 2). ( c ) RRN3 interacts with Top2α of Pol Iβ in far-western analysis. Pol Iα and Iβ were probed with 35 S-Flag-RRN3 and Top2α-antibodies. ( d ) Top2α C-terminus is important for RRN3 interaction. In vitro -translated and Flag-immunopurified 35 S-Flag-RRN3 was incubated with in vitro -translated 35 S-GFP-Top2α WT and C-terminal-truncated (st5; 180 amino-acid deletion) proteins on GFP-antibody beads. Input RRN3 (1%, lane 1); RRN3 with GFP-antibody beads (lane 4); *contaminating translation product. ( e ) Efficient co-IP of Top2α with Pol Iβ requires its C-terminal 42 amino acids. Top2α was immunoprecipitated from HTETOP cells depleted for endogenous Top2α and stably expressing GFP-Top2α-WT and C-terminal-truncated (st1, 42 amino-acid deletion) proteins, using GFP antibodies. IgG control (lane 1). Immunoprecipitates were immunoblotted using antibodies for Top2α, PAF53 and RRN3. Representative immunoblot is shown. Quantitation and normalization of the RRN3 and PAF53 immunoblot signals to those of Top2α-WT and -st1, in three independent experiments, revealed that C-terminal 42 amino-acid truncation of Top2α reduced RRN3 and PAF53 signals ~sixfold and ~twofold, respectively. ( f ) Top2α occupancy of the rDNA promoter is reduced in TAF I 41-depleted cells with decreased rRNA transcription. HEK293 cells were transfected with scrambled or SL1 subunit TAF I 41 (TAF1D) small interfering RNAs (siRNAs). rDNA-promoter occupancy by Top2α, Pol I subunit A135 and SL1 subunit TAF I 110 (TAF1C) in these cells was analysed by ChIP using Top2α, A135 and TAF I 110 antibodies; data in bar graphs are from three independent ChIP experiments, normalized to control IgG samples; s.d. is shown. ( g ) Control for f showing pre-rRNA levels from cells transfected with scrambled siRNA (lane 1) or TAF I 41 siRNA (lane 2) as analysed by S1 nuclease protection. Full size image To substantiate an association of Top2α with Pol Iβ in cells, we immunoprecipitated Pol I from nuclear extracts of HeLa cells transiently expressing Flag-tagged Pol I subunit CAST [32] , using Flag-specific antibodies, then immunoblotted the immunoprecipitates using antibodies specific for Top2α, RRN3 and Pol I subunits PAF53 and AC19. Top2α co-immunoprecipitated with Pol I in this experiment ( Fig. 1b ). We also passed purified Pol Iβ over a Top2α-antibody column and analysed proteins eluted from the column and proteins in the flow-through in immunoblot and promoter-specific transcription assays ( Supplementary Fig. S1b–d ). Intriguingly, the majority of promoter-specific transcription activity was lost and most of the RRN3 protein was depleted from Pol Iβ and retained on the Top2α-antibody column. Therefore, the specific Top2α antibody used disrupted Top2α and RRN3 interactions with Pol I. These data indicate that the majority of Pol Iβ complexes purified from human cell nuclei include Top2α. Top2α interacts directly with Pol Iβ-specific component RRN3 We reasoned that a direct interaction between Top2α and Pol Iβ might involve Pol Iβ-specific component RRN3. Two polypeptides unique to Pol Iβ bound to RRN3, the larger of which migrated similarly to full-length Top2α protein, in a Far-western analysis in which in vitro -translated 35 S-labelled hRRN3 was used to probe renatured Pol Iα or Pol Iβ ( Fig. 1c ). Moreover, there was a direct interaction between RRN3 and Top2α in a recombinant protein-binding assay, in which in vitro -translated RRN3 was incubated with in vitro -translated green fluorescent protein (GFP)-Top2α [33] on GFP-antibody beads ( Fig. 1d ). To test the likely involvement of the isoform-specific CTD in the interaction of Top2α with RRN3, we used Top2α CTD-mutant proteins lacking the terminal 42 or 180 amino acids (st1 or st5, respectively). These were the shortest and longest of a series of CTD truncations shown to impair the ability of GFP-Top2α to rescue the conditional Top2α-mutant cell line HTETOP [33] from lethal Top2α depletion ( Supplementary Fig. S2 ). A C-terminal-truncated version of Top2α (st5, 180 amino-acid deletion) displayed significantly reduced interaction with RRN3 in the recombinant protein-binding assay ( Fig. 1d ). To further assess Top2α–RRN3 interactions, nuclear extracts of HTETOP cells depleted of endogenous Top2α [33] and stably expressing GFP-Top2α-wild type (WT) or -st1 (CTD 42 amino-acid deletion) were incubated with GFP-specific antibodies, and immunoprecipitates were immunoblotted using antibodies specific for Top2α, RRN3 and Pol I subunit PAF53. Endogenous RRN3 and Pol I subunit PAF53 co-immunoprecipitated with GFP-Top2α-WT ( Fig. 1e ). There was a significant decrease (~sixfold) in the amount of RRN3 that co-immunoprecipitated with the GFP-Top2α-st1 mutant, compared with GFP-Top2α-WT. There was also a decrease (~twofold) in the amount of PAF53 co-immunoprecipitated; the smaller magnitude of this decrease might reflect interactions between Top2α and other components of the initiation-competent Pol Iβ complex, such as CK2 [23] . Collectively, these data demonstrate that Top2α interacts directly with RRN3 and that residues 1491-1531 in the Top2α CTD are important for such interaction. Therefore, there is evidence, both in vitro and in cells, to support an interaction between Top2α and RRN3 as components of initiation-competent Pol Iβ. Top2α occupies the rDNA promoter in an SL1-dependent manner The association of Top2α with initiation-competent Pol Iβ predicts the presence of Top2α at the rDNA promoter. Top2α was detectable at the rDNA promoter by chromatin immunoprecipitation (ChIP) analysis in all cell types tested ( Fig. 1f and Supplementary Fig. S3 ); elsewhere, along the rDNA repeat, Top2α association varied according to cell type ( Supplementary Fig. S3 ). Small interfering RNA-mediated depletion of the TAF I 41 subunit of SL1 in cells, which leads to the disappearance of SL1 and Pol I from the rDNA promoter and reduces Pol I transcription [34] , resulted in the loss of Top2α from the rDNA promoter ( Fig. 1f and g ). The data suggest that SL1, which binds to the rDNA promoter and recruits Pol Iβ through RRN3, is required for the recruitment of Top2α to the rDNA promoter in cells and that the presence of Top2α at the rDNA promoter correlates with the presence of Pol Iβ and Pol I transcription. Top2α and RRN3 dissociate from Pol I following initiation RRN3 dissociates from Pol I at an early step following initiation of transcription [35] , [36] , and we have used a stalled Pol I transcription system [37] to assess whether Top2α and RRN3 both dissociate from Pol I following initiation of transcription. Pol I can be stalled at the position of the first T (+31) on a ‘T-less’ template when the transcription reaction is carried out in the absence of UTP. Immobilization of the template allows the template-associated proteins to be separated from proteins that dissociate from the transcription complex after initiation of transcription. We demonstrate that Pol I subunit PAF53 was still associated with the DNA template following initiation of transcription, as expected for a stalled Pol I complex ( Fig. 2a , lane 1), whereas RRN3 and Top2α were present in the reaction supernatant ( Fig. 2a , lane 2). Note that in control transcription reactions supplemented with all four NTPs, Pol I transcribes to the end of the template, whereupon it dissociates in the presence of excess competitor DNA ( Fig. 2a , lane 3) and, consequently, Pol I and Pol I-associated factors were present in the reaction supernatant ( Fig. 2a , lane 4). Therefore, both Top2α and RRN3 dissociate from Pol I following initiation of transcription in vitro ( Fig. 2b ), consistent with a tethering of Top2α to Pol I, at least in part, through RRN3. Should Top2α indeed dissociate from Pol I at initiation or during/immediately following promoter escape in cells, any role for Pol Iβ-associated Top2α in Pol I transcription would be predicted to be at an early step in transcription. 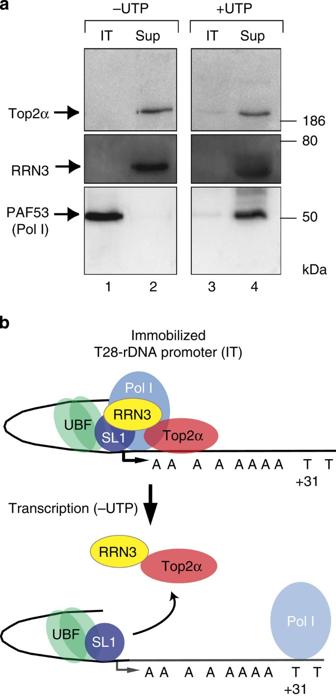Figure 2: Top2α and RRN3 dissociate from the Pol Iβ complex following transcription initiationin vitro. (a) Using purified Pol Iβ, SL1 and UBF, PICs were assembled at the rDNA promoter of an immobilized T-less template ‘T28’ (IT)37. Transcription reactions were performed in the presence of ATP, GTP and CTP (−UTP, left panel) or all four NTPs (+UTP, right panel). Excess competitor DNA was added to transcription reactions to prevent re-association of factors with template. After completion of transcription, the reaction mix (Sup) was separated from the template (IT), which was then washed. Proteins bound to the template (lanes 1 and 3) and proteins released from the template into the reaction mix during transcription (Sup lanes 2 and 4) were subjected to SDS–PAGE and immunoblotting using antibodies to Top2α, RRN3 and PAF53. (b) Schematic interpretation of results. Figure 2: Top2α and RRN3 dissociate from the Pol Iβ complex following transcription initiation in vitro . ( a ) Using purified Pol Iβ, SL1 and UBF, PICs were assembled at the rDNA promoter of an immobilized T-less template ‘T28’ (IT) [37] . Transcription reactions were performed in the presence of ATP, GTP and CTP (−UTP, left panel) or all four NTPs (+UTP, right panel). Excess competitor DNA was added to transcription reactions to prevent re-association of factors with template. After completion of transcription, the reaction mix (Sup) was separated from the template (IT), which was then washed. Proteins bound to the template (lanes 1 and 3) and proteins released from the template into the reaction mix during transcription (Sup lanes 2 and 4) were subjected to SDS–PAGE and immunoblotting using antibodies to Top2α, RRN3 and PAF53. ( b ) Schematic interpretation of results. Full size image Effects of Top2 inhibition on Pol I transcription To investigate a role for Top2α in early Pol I transcription events, we first tested the effects of inhibition of Top2 activity on Pol I transcription, using 3 H-uridine pulse-chase labelling of (pre-)rRNA in cells. We observed a negative effect on Pol I transcription of etoposide treatment of U2OS cells ( Supplementary Fig. S4 ). However, there is evidence to suggest that this was likely to be indirect and as a consequence of ataxia telangiectasia mutated (ATM)- [38] and p53-dependent DNA-damage signaling [39] , [40] , activated by double-strand DNA breaks arising from trapped Top2–DNA cleavage complexes [1] . Therefore, to assess whether inhibition of Top2 activity could induce any effects on Pol I transcription independent of DNA-damage signalling, we treated cells with alternative Top2 inhibitors and/or used cell lines that could not elicit a p53-dependent DNA-damage response. Crucially, treatment for up to 15 h of U2OS cells with merbarone (a Top2 catalytic inhibitor blocking DNA cleavage [41] ) and of p53-null H1299 cells with etoposide ( Fig. 3a–c ) produced no significant effects on Pol I transcription. As inhibition of Top2 activity for up to 15 h does not have a detectable direct effect on Pol I transcription in actively growing cell populations, this suggests that Top2 activity is not essential for transcription (re-)initiation or elongation of rRNA transcripts. Notably, Top2 inhibitor treatments for 24 and 48 h, of U2OS cells with merbarone or HCT116 (p53 null) cells with etoposide, resulted in significant decreases in Pol I transcription ( Fig. 3d–f ). These findings imply a potential role for Top2 in Pol I transcription, outside of (re-)initiation or elongation. 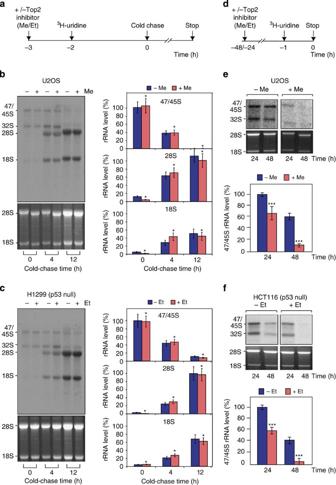Figure 3: Effects of Top2 inhibition on Pol I transcription. (a) Schematic of pulse-chase labelling of cells with3H-uridine to determine effects of Top2 inhibition on rRNA synthesis by Pol I (used inbandc) (b) Pre-rRNA (47/45S), 28S and 18S rRNA transcript levels in actively growing U2OS cells were unaffected by treatment with Top2 inhibitor merbarone (Me) for up to 15 h.3H-uridine was added 1 h after Me; non-radioactive uridine was added after an additional 2 h. Total RNA was extracted after 0, 4 and 12 h, separated by formaldehyde agarose gel electrophoresis and transferred to membrane. Newly synthesized pre-rRNA and rRNA transcripts were detected by autoradiography (representative experiment; upper panel); total 18S and 28S rRNAs were detected by ethidium bromide staining (lower panel). Relative efficiencies of rRNA synthesis and transcript processing are shown (bar graphs: −Me, dark-blue bars;+Me, light-red bars) for 47S/45S pre-rRNA (top), 28S rRNA (middle) and 18S rRNA (bottom), expressed as percentage of highest value (set at 100%). s.d. is shown,n=3; *P<0.05. (c) Pre-rRNA (47/45S), 28S and 18S rRNA transcript levels in actively growing H1299 cells (p53 null) were unaffected by treatment with etoposide (Et) for up to 15 h. Experimental details as inaandb, except H1299 instead of U2OS cells; Et instead of Me. (d) Schematic of3H-uridine labelling of cells to determine effects of Top2 inhibition on rRNA synthesis (used ineandf). (e) Pre-rRNA (47/45S) and 32S rRNA transcript levels in actively growing U2OS cells were reduced by treatment with Me for 24 or 48 h. Newly synthesized pre-rRNA and rRNA transcripts from cells treated with Me for 24 or 48 h, then incubated with3H-uridine for 1 h, were detected, quantitated and expressed as inb: representative experiment (upper panel); total 18S and 28S rRNAs (lower panel); and 47S/45S pre-rRNA bar graphs (−Me, dark-blue bars;+Me, light-red bars). s.d. is shown,n=3; ***P<0.001. (f) Pre-rRNA (47/45S) and 32S rRNA transcript levels in HCT116 (p53 null) cells were reduced by treatment with Et for 24 or 48 h. Experimental details as ine. Figure 3: Effects of Top2 inhibition on Pol I transcription. ( a ) Schematic of pulse-chase labelling of cells with 3 H-uridine to determine effects of Top2 inhibition on rRNA synthesis by Pol I (used in b and c ) ( b ) Pre-rRNA (47/45S), 28S and 18S rRNA transcript levels in actively growing U2OS cells were unaffected by treatment with Top2 inhibitor merbarone (Me) for up to 15 h. 3 H-uridine was added 1 h after Me; non-radioactive uridine was added after an additional 2 h. Total RNA was extracted after 0, 4 and 12 h, separated by formaldehyde agarose gel electrophoresis and transferred to membrane. Newly synthesized pre-rRNA and rRNA transcripts were detected by autoradiography (representative experiment; upper panel); total 18S and 28S rRNAs were detected by ethidium bromide staining (lower panel). Relative efficiencies of rRNA synthesis and transcript processing are shown (bar graphs: −Me, dark-blue bars;+Me, light-red bars) for 47S/45S pre-rRNA (top), 28S rRNA (middle) and 18S rRNA (bottom), expressed as percentage of highest value (set at 100%). s.d. is shown, n =3; * P <0.05. ( c ) Pre-rRNA (47/45S), 28S and 18S rRNA transcript levels in actively growing H1299 cells (p53 null) were unaffected by treatment with etoposide (Et) for up to 15 h. Experimental details as in a and b , except H1299 instead of U2OS cells; Et instead of Me. ( d ) Schematic of 3 H-uridine labelling of cells to determine effects of Top2 inhibition on rRNA synthesis (used in e and f ). ( e ) Pre-rRNA (47/45S) and 32S rRNA transcript levels in actively growing U2OS cells were reduced by treatment with Me for 24 or 48 h. Newly synthesized pre-rRNA and rRNA transcripts from cells treated with Me for 24 or 48 h, then incubated with 3 H-uridine for 1 h, were detected, quantitated and expressed as in b : representative experiment (upper panel); total 18S and 28S rRNAs (lower panel); and 47S/45S pre-rRNA bar graphs (−Me, dark-blue bars;+Me, light-red bars). s.d. is shown, n =3; *** P <0.001. ( f ) Pre-rRNA (47/45S) and 32S rRNA transcript levels in HCT116 (p53 null) cells were reduced by treatment with Et for 24 or 48 h. Experimental details as in e . Full size image Top2α depletion negatively affects Pol Iβ assembly/stability To further explore the possibility of a role for Top2α in Pol I transcription, we analysed rRNA transcripts from HTETOP cells specifically depleted of the α-isoform of Top2 by treatment with tetracycline (Tet) for 48 h ( Fig. 4a and b ). In common with other cells depleted of Top2α protein or treated with Top2 catalytic inhibitors (reviewed in Nitiss [1] ), this impairs sister chromatid segregation causing aberrant anaphases and cytokinesis [16] , [33] . After 48 h in Tet, the only mRNA transcripts to be dramatically depleted in HTETOP cells are those encoding Top2α itself [42] . Nevertheless, we detected an ~twofold reduction in Pol I synthesis of the 47S pre-rRNA transcript, with no effect on pre-rRNA processing ( Fig. 4c ). Pol I was immunoprecipitated from the Top2α-depleted and control cells in equivalent amounts, as determined by the non-specific Pol I transcription activities of the immunoprecipitates ( Fig. 4d ). Yet, there was significantly less promoter-specific transcription activity associated with Pol I immunoprecipitates from the Top2α-depleted cells ( Fig. 4d ) and a reduced amount of RRN3 protein in these immunoprecipitates ( Fig. 4e ), compared with those of the control cells. These data suggest the presence of fewer initiation-competent Pol Iβ complexes in Top2α-depleted cells. Such a decrease could account for the observed two-fold reduction in Pol I transcription in Top2α-depleted cells. Taken together, these results suggest that Top2α can influence the assembly and/or stability of initiation-competent Pol Iβ at the rDNA promoter, and thereby PIC formation, in cells. 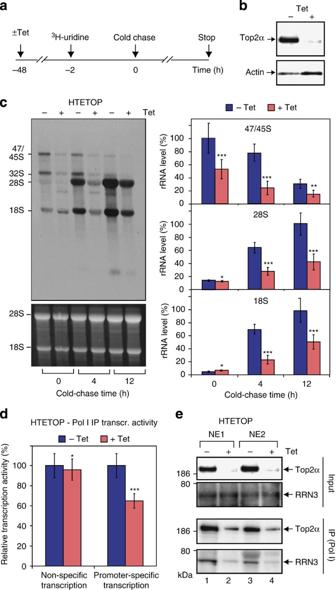Figure 4: Top2α depletion downregulates Pol I transcription and the level of the initiation-competent Pol Iβ complex in cells. (a) Schematic of3H-uridine pulse-chase labelling of cells to determine effects of Top2α depletion on rRNA synthesis (used inc). (b) Control for Top2α-depletion. HTETOP cells33were incubated for 48 h with 1 μg ml−1Tet (+Tet) or without (−Tet). Proteins were immunoblotted using Top2α and actin antibodies. (c) rRNA synthesis is reduced in Top2α-depleted cells. Cells depleted of Top2α, as inb, were3H-uridine labelled for 2 h and cold-chased with uridine, and RNA was extracted after 0, 4 and 12 h. Newly synthesized transcripts were detected by autoradiography (representative experiment; upper panel); 18S and 28S rRNAs were ethidium bromide stained (lower panel). Relative efficiencies of rRNA synthesis and transcript processing are shown (bar graphs: −Tet, dark-blue bars;+Tet, light-red bars) for 47S/45S pre-rRNA (top), 28S rRNA (middle) and 18S rRNA (bottom), expressed as percentage of highest value (set at 100%). s.d. is shown,n=3; ***P<0.001, **P<0.01 and *P<0.05. (d) Pol I from Top2α-depleted cells supports a reduced level of rDNA promoter-specific Pol I transcription activity. HTETOP cells, transfected with Flag-CAST (Pol I subunit), were incubated with or without Tet for 48 h. Pol I complexes immunoprecipitated using Flag-antibody were analysed for non-specific transcription activity and rDNA promoter-specific transcription activity in a run-off transcription assay. Relative levels of non-specific and promoter-specific transcription in Top2α-depleted (+Tet, light-red bars) or non-depleted (−Tet, dark-blue bars) cells are indicated in the graph. s.d. is shown,n=3; ***P<0.001 and *P<0.05. The non-specific transcription activities of Pol I immunoprecipitated from Tet− and Tet+ cells were similar, reflecting that similar amounts of Pol I were immunoprecipitated. (e) The amount of RRN3 co-immunoprecipitating with Pol I is reduced in Top2α-depleted cells. Pol I complexes, immunoprecipitated from nuclear extracts of Flag-CAST-transfected HTETOP cells incubated with (+Tet) or without Tet (−Tet) for 48 h, were analysed by immunoblotting, using Top2α and RRN3 antibodies. Immunoblots of the nuclear extract inputs (upper panels) and Pol I immunoprecipitates (lower panels) from two independent experiments (NE1 and NE2) are shown. Figure 4: Top2α depletion downregulates Pol I transcription and the level of the initiation-competent Pol Iβ complex in cells. ( a ) Schematic of 3 H-uridine pulse-chase labelling of cells to determine effects of Top2α depletion on rRNA synthesis (used in c ). ( b ) Control for Top2α-depletion. HTETOP cells [33] were incubated for 48 h with 1 μg ml −1 Tet (+Tet) or without (−Tet). Proteins were immunoblotted using Top2α and actin antibodies. ( c ) rRNA synthesis is reduced in Top2α-depleted cells. Cells depleted of Top2α, as in b , were 3 H-uridine labelled for 2 h and cold-chased with uridine, and RNA was extracted after 0, 4 and 12 h. Newly synthesized transcripts were detected by autoradiography (representative experiment; upper panel); 18S and 28S rRNAs were ethidium bromide stained (lower panel). Relative efficiencies of rRNA synthesis and transcript processing are shown (bar graphs: −Tet, dark-blue bars;+Tet, light-red bars) for 47S/45S pre-rRNA (top), 28S rRNA (middle) and 18S rRNA (bottom), expressed as percentage of highest value (set at 100%). s.d. is shown, n =3; *** P <0.001, ** P <0.01 and * P <0.05. ( d ) Pol I from Top2α-depleted cells supports a reduced level of rDNA promoter-specific Pol I transcription activity. HTETOP cells, transfected with Flag-CAST (Pol I subunit), were incubated with or without Tet for 48 h. Pol I complexes immunoprecipitated using Flag-antibody were analysed for non-specific transcription activity and rDNA promoter-specific transcription activity in a run-off transcription assay. Relative levels of non-specific and promoter-specific transcription in Top2α-depleted (+Tet, light-red bars) or non-depleted (−Tet, dark-blue bars) cells are indicated in the graph. s.d. is shown, n =3; *** P <0.001 and * P <0.05. The non-specific transcription activities of Pol I immunoprecipitated from Tet− and Tet+ cells were similar, reflecting that similar amounts of Pol I were immunoprecipitated. ( e ) The amount of RRN3 co-immunoprecipitating with Pol I is reduced in Top2α-depleted cells. Pol I complexes, immunoprecipitated from nuclear extracts of Flag-CAST-transfected HTETOP cells incubated with (+Tet) or without Tet (−Tet) for 48 h, were analysed by immunoblotting, using Top2α and RRN3 antibodies. Immunoblots of the nuclear extract inputs (upper panels) and Pol I immunoprecipitates (lower panels) from two independent experiments (NE1 and NE2) are shown. Full size image We reasoned that in a population of actively growing cells, at any one time, most of the active rDNA promoters are engaged in multiple-round transcription, with relatively few requiring de novo PIC formation and activation of transcription. De novo PIC formation is required at actively transcribing rDNA genes following DNA replication (on one set of duplicates). Lack of de novo PIC assembly would lead to a predicted ~50% reduction in Pol I transcription with each cell cycle. Our data ( Figs 3 and 4 ) suggest that in the absence of Top2α activity, there may be a gradual accumulation of rDNA promoters requiring de novo PIC formation to achieve transcription. Top2α facilitates assembly of Pol I PICs To investigate the involvement of Top2α in de novo PIC formation, we sought a system in which de novo functional PIC formation was required for Pol I transcription at the majority of rDNA promoters. Pol I transcription can be downregulated by serum starvation of cells and activated by serum refeeding [43] , [44] . Starved U2OS cells exhibit decreased levels of Pol I transcription ( Fig. 5a ), accompanied by reduction of SL1 and Pol I from the rDNA promoter ( Fig. 5b ) and the disappearance of Top2α from the rDNA promoter (as determined by ChIP) ( Fig. 5b ) and the nucleolus (as determined by indirect immunofluorescence; Supplementary Fig. S5 ). Activation of Pol I transcription occurs in starved H1299, U2OS and HTETOP cells following serum refeeding ( Fig. 6a–c , respectively). This activation correlates with an increase in SL1, UBF and Pol I promoter occupancies and the reappearance of Top2α at the rDNA promoter ( Fig. 6d ), as well as increased Top2α expression and co-localisation of Top2α with Pol I in the nucleolus ( Fig. 6f and Supplementary Fig. S5b ). Therefore, de novo functional PIC formation appears to be required for transcription at the majority of rDNA promoters re-activated in serum-refed cells. There are several hundred copies of the rRNA genes per cell, but only about half are active in cycling cells and sensitive to psoralen cross-linking, and these are in an open chromatin configuration. Despite the changes in Pol I transcription caused by starvation or growth-stimulation of cells, the proportion of rRNA genes in an open chromatin configuration remains constant [43] , [45] . This suggests that the rRNA genes requiring de novo PIC formation for activation upon serum refeeding are likely to be from the pool of genes sensitive to psoralen cross-linking. We exploited this system to investigate the requirement for Top2α in de novo PIC formation in Pol I transcription. 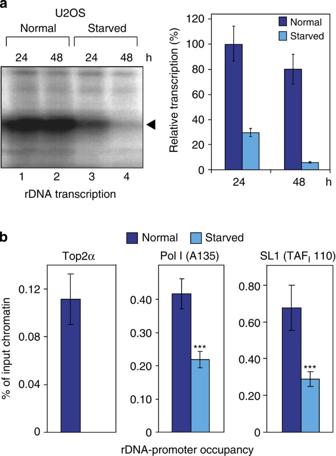Figure 5: Serum-starvation induced downregulation of Pol I transcription is accompanied by reduced SL1 and Pol I and loss of Top2α at the rDNA promoter. (a) rDNA transcription decreases upon starvation of U2OS cells. Total RNA was extracted from actively growing U2OS cells (normal, lanes 1 and 2 of panel; dark-blue bars in graph) or from U2OS cells serum-starved for 24 or 48 h (starved, lanes 3 and 4 of panel; light-blue bars in graph). Pre-rRNA levels were analysed by S1 nuclease protection analysis using a probe hybridizing to the first 40 nucleotides of the pre-rRNA. (b) SL1, Pol I and Top2α occupancies of the rDNA promoter are reduced in starved cells. ChIP analysis of the rDNA-promoter region of actively growing U2OS cells (normal, dark-blue bars) or U2OS cells starved of serum for 20 h (starved, light-blue bars), using antibodies specific for Top2α, Pol I subunit A135 and SL1 subunit TAFI110 (TAF1C). s.d. is shown,n=3; ***P<0.001. Figure 5: Serum-starvation induced downregulation of Pol I transcription is accompanied by reduced SL1 and Pol I and loss of Top2α at the rDNA promoter. ( a ) rDNA transcription decreases upon starvation of U2OS cells. Total RNA was extracted from actively growing U2OS cells (normal, lanes 1 and 2 of panel; dark-blue bars in graph) or from U2OS cells serum-starved for 24 or 48 h (starved, lanes 3 and 4 of panel; light-blue bars in graph). Pre-rRNA levels were analysed by S1 nuclease protection analysis using a probe hybridizing to the first 40 nucleotides of the pre-rRNA. ( b ) SL1, Pol I and Top2α occupancies of the rDNA promoter are reduced in starved cells. ChIP analysis of the rDNA-promoter region of actively growing U2OS cells (normal, dark-blue bars) or U2OS cells starved of serum for 20 h (starved, light-blue bars), using antibodies specific for Top2α, Pol I subunit A135 and SL1 subunit TAF I 110 (TAF1C). s.d. is shown, n =3; *** P <0.001. 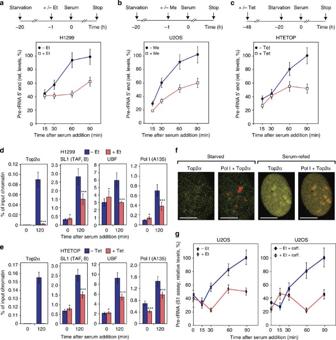Figure 6: Top2α facilitates formation of PICs in Pol I transcription activation. (a,b) Top2 inhibition reduces activation of Pol I transcription in serum-refed cells. H1299 cells (p53 null) (a) or U2OS cells (b) were serum-starved for 20 h and (starting at –1 h) incubated with Top2 inhibitors etoposide (Et) or merbarone (Me), respectively, or without inhibitors, for 1 h. At 0 h, serum was added to the cells. RNA was extracted 15, 30, 60 and 90 min after serum addition. Pre-rRNA levels were analysed by S1 nuclease protection (complementary assay,3H-uridine labelling of RNA,Supplementary Fig. S6a,b); s.d. is shown. (c) Top2α depletion reduces activation of Pol I transcription in serum-refed cells. HTETOP cells were incubated for 48 h +/− Tet, with serum starvation for the last 20 h. Serum was added back and Pol I transcription assayed as ina(complementary assay,Supplementary Fig. S6c). (d,e) Inhibition of Top2 or depletion of Top2α reduces the accumulation of PIC components SL1, UBF and Pol I at the rDNA promoter in serum-refed cells. ChIP assays were performed on chromatin from cells treated as inaandc, respectively, using antibodies for Top2α, TAFI63 (TAF1B; SL1), UBF and A135 (Pol I), and normalized to control IgG samples. s.d. is shown,n=3; ***P<0.001 and *P<0.05. (f) Top2α co-localises with Pol I upon activation of Pol I transcription. U2OS cells serum-starved for 20 h were serum-refed for 2 h, then analysed by indirect immunofluorescence, using antibodies for A194 (Pol I; red) or Top2α (green), and laser scanning confocal microscopy. Scale bar, 10.4 μm (expanded version,Supplementary Fig. S5b). (g) The reduction in activation of Pol I transcription detected in serum-refed cells treated with Top2 inhibitor is not affected by treatment with caffeine, an inhibitor of ATM/ATR. U2OS cells were serum-starved (20 h) and incubated with or without Et (25 μM) and without (left panel) or with caffeine (125 μM) (right panel) 1 h before addition of serum. RNA was extracted at 0, 15, 30, 60 and 90 min following serum addition, and pre-rRNA levels were analysed as ina. Full size image Figure 6: Top2α facilitates formation of PICs in Pol I transcription activation. ( a , b ) Top2 inhibition reduces activation of Pol I transcription in serum-refed cells. H1299 cells (p53 null) ( a ) or U2OS cells ( b ) were serum-starved for 20 h and (starting at –1 h) incubated with Top2 inhibitors etoposide (Et) or merbarone (Me), respectively, or without inhibitors, for 1 h. At 0 h, serum was added to the cells. RNA was extracted 15, 30, 60 and 90 min after serum addition. Pre-rRNA levels were analysed by S1 nuclease protection (complementary assay, 3 H-uridine labelling of RNA, Supplementary Fig. S6a,b ); s.d. is shown. ( c ) Top2α depletion reduces activation of Pol I transcription in serum-refed cells. HTETOP cells were incubated for 48 h +/− Tet, with serum starvation for the last 20 h. Serum was added back and Pol I transcription assayed as in a (complementary assay, Supplementary Fig. S6c ). ( d , e ) Inhibition of Top2 or depletion of Top2α reduces the accumulation of PIC components SL1, UBF and Pol I at the rDNA promoter in serum-refed cells. ChIP assays were performed on chromatin from cells treated as in a and c , respectively, using antibodies for Top2α, TAF I 63 (TAF1B; SL1), UBF and A135 (Pol I), and normalized to control IgG samples. s.d. is shown, n =3; *** P <0.001 and * P <0.05. ( f ) Top2α co-localises with Pol I upon activation of Pol I transcription. U2OS cells serum-starved for 20 h were serum-refed for 2 h, then analysed by indirect immunofluorescence, using antibodies for A194 (Pol I; red) or Top2α (green), and laser scanning confocal microscopy. Scale bar, 10.4 μm (expanded version, Supplementary Fig. S5b ). ( g ) The reduction in activation of Pol I transcription detected in serum-refed cells treated with Top2 inhibitor is not affected by treatment with caffeine, an inhibitor of ATM/ATR. U2OS cells were serum-starved (20 h) and incubated with or without Et (25 μM) and without (left panel) or with caffeine (125 μM) (right panel) 1 h before addition of serum. RNA was extracted at 0, 15, 30, 60 and 90 min following serum addition, and pre-rRNA levels were analysed as in a . Full size image There was a marked (~twofold) reduction in activation of Pol I transcription in starved H1299 and U2OS cells treated with Top2 inhibitors etoposide and merbarone, respectively, then resupplied with serum, as determined by S1 nuclease protection of the first 40 nucleotides of the pre-rRNA ( Fig. 6a ) and by 3 H-uridine pulse-chase labelling ( Supplementary Fig. S6a,b ). Top2 inhibitor ICRF-193 similarly reduced activation of Pol I transcription in U2OS cells ( Supplementary Fig. S6d,e ). These data suggested a defect in the early stages of transcription. There was a corresponding reduced occupancy of SL1, UBF and Pol I, with little Top2α detectable, at the rDNA promoter in the H1299 cells ( Fig. 6d ), suggesting that, inhibition of Top2 activity reduces the efficiency of PIC formation and, thereby, the efficiency of Pol I transcription activation. This defect in activation is likely to be independent of DNA-damage signalling through p53 and ATM as it occurred in p53-null cells (H1299) ( Fig. 6a ) and could not be rescued by incubation of cells with caffeine (an inhibitor of ATM/ATR [ataxia telangiectasia and Rad3-related] signalling) ( Fig. 6g ). HTETOP cells depleted of Top2α protein, serum-starved, then resupplied with serum, also showed reduced activation of Pol I transcription and a corresponding reduced promoter occupancy of SL1, UBF and Pol I ( Fig. 6c and Supplementary Fig. S6c ), complementing the results obtained by pharmacological inhibition of Top2. Taken together, these results suggest that Top2 activity, specifically that of the α-isoform of Top2, facilitates the efficient de novo assembly of PICs in Pol I transcription. Top2α induces DNA cleavage at the rDNA promoter in activation We hypothesized that Top2α might influence de novo PIC formation in activation of Pol I transcription by producing topological changes at the rDNA promoter that would support efficient assembly of the PIC. We reasoned that double-strand DNA (dsDNA) cleavage would arise at the rDNA promoter from such Top2 activity, although short-lived, due to the re-ligation activity of Top2. Therefore, we analysed the rDNA-promoter region for DNA breaks. To this end, cells were fixed and permeabilized at different time points following serum refeeding, incubated with biotin-11–deoxyuridine triphosphate (dUTP) and deoxynucleotide transferase (TdT) to label DNA breaks, and then, DNA containing breaks was captured on streptavidin beads and analysed by qPCR, as described [19] . Strikingly, a significant increase in DNA cleavage at the rDNA promoter was detectable during the activation of Pol I transcription ( Fig. 7a ). The time course demonstrates that the DNA cleavage is transient, peaking at the first detection of transcription activation and Top2α occupancy of the rDNA promoter. Importantly, no such DNA cleavage was detectable at the rDNA promoter in the Top2α-depleted and starved HTETOP cells upon serum refeeding ( Fig. 7b ). Note that although enhanced DNA cleavage has been observed at other regions of the rDNA in some experiments upon serum refeeding and Pol I transcription activation, this was not a reproducible effect. In other control experiments, we did not observe any increase in DNA cleavage at the promoters of the glyceraldehyde-3-phosphate dehydrogenase and peptidylprolyl isomerase A genes upon serum refeeding ( Supplementary Fig. S7 ). 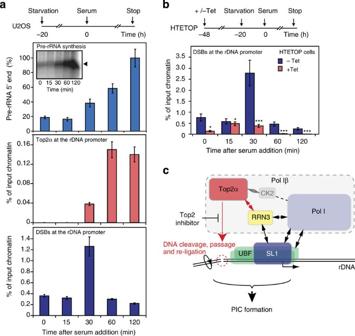Figure 7: Top2α activity is required for the transient appearance of double-strand DNA breaks in the rDNA-promoter region occurring upon Pol I transcription activation. (a) Transient double-strand DNA breaks (DSBs) occur in the rDNA-promoter region upon activation of Pol I transcription. Pre-rRNA levels (S1 nuclease protection assay in insert of graph, top panel), Top2α occupancy (ChIP, middle panel) and DSBs (bottom panel) of the rDNA-promoter region were analysed 0, 15, 30, 60 and 120 min after add-back of serum to U2OS cells serum-starved for 20 h. s.d. is shown,n=3. (b) Top2α depletion abrogates transient DSBs. HTETOP cells were incubated for 48 h with Tet (+Tet; resulting in Top2α depletion) or without (−Tet), with serum starvation for the last 20 h. DSBs at the rDNA-promoter region (promoter primer pair, seeSupplementary Table S3, covered −56 to +17 relative to the transcription start site at +1; the chromatin had been sonicated to an average fragment size of ~300 bp) were analysed 0, 15, 30, 60 and 120 min after add-back of serum to the cells. s.d. is shown,n=3; ***P<0.001 and *P<0.05. (c) The schematic shows the interactions of Top2α with other RNA Pol I transcription components at the rDNA promoter and a model in which transient Top2α-mediated double-strand DNA cleavage, passage and re-ligation in the rDNA-promoter region changes the DNA topology (indicated by a ‘swivel’) to facilitatede novoPIC formation in activation of Pol I transcription. Figure 7: Top2α activity is required for the transient appearance of double-strand DNA breaks in the rDNA-promoter region occurring upon Pol I transcription activation. ( a ) Transient double-strand DNA breaks (DSBs) occur in the rDNA-promoter region upon activation of Pol I transcription. Pre-rRNA levels (S1 nuclease protection assay in insert of graph, top panel), Top2α occupancy (ChIP, middle panel) and DSBs (bottom panel) of the rDNA-promoter region were analysed 0, 15, 30, 60 and 120 min after add-back of serum to U2OS cells serum-starved for 20 h. s.d. is shown, n =3. ( b ) Top2α depletion abrogates transient DSBs. HTETOP cells were incubated for 48 h with Tet (+Tet; resulting in Top2α depletion) or without (−Tet), with serum starvation for the last 20 h. DSBs at the rDNA-promoter region (promoter primer pair, see Supplementary Table S3 , covered −56 to +17 relative to the transcription start site at +1; the chromatin had been sonicated to an average fragment size of ~300 bp) were analysed 0, 15, 30, 60 and 120 min after add-back of serum to the cells. s.d. is shown, n =3; *** P <0.001 and * P <0.05. ( c ) The schematic shows the interactions of Top2α with other RNA Pol I transcription components at the rDNA promoter and a model in which transient Top2α-mediated double-strand DNA cleavage, passage and re-ligation in the rDNA-promoter region changes the DNA topology (indicated by a ‘swivel’) to facilitate de novo PIC formation in activation of Pol I transcription. Full size image Our data imply that, in activation of Pol I transcription, Top2α, specifically, induces the transient appearance of double-strand DNA breaks in the rDNA-promoter region, reflecting its dsDNA cleavage, strand passage and re-ligation activity. Taken together, the data suggest that Top2α activity at the rDNA promoter facilitates the efficient de novo assembly of functional PICs, which include SL1, UBF and Pol Iβ ( Fig. 7c ). This study identifies a novel function for a Top2 in facilitating de novo PIC formation and activation of Pol I transcription of the rRNA genes in human cells. We present evidence of a role for the Top2α isoform in Pol I transcription. Our data suggest that active Top2α is a component of the initiation-competent Pol Iβ complex, targeted to the rDNA promoter, at least in part, through the interaction of its isoform-specific C terminus with the RRN3 component of Pol Iβ, which interacts with promoter-bound transcription factor SL1. Depletion of Top2α negatively affects the assembly and/or stability of initiation-competent Pol Iβ and decreases Pol I transcription in cells, implying that Top2α can influence the assembly and/or stability of initiation-competent Pol Iβ at the rDNA promoter and, thereby, PIC formation in cells. De novo PIC formation is an event expected to occur at the active rDNA gene promoters following DNA replication (on one set of the duplicates) during each cell cycle. De novo functional PIC formation is also required for activation of Pol I transcription at the majority of rDNA promoters upon refeeding of serum-starved cells, and we discovered that Top2α facilitates efficient activation of Pol I transcription from such promoters and that this is accompanied by Top2α-dependent DNA cleavage and accumulation of PIC components and Top2α at the rDNA-promoter region. Our data suggest a role for Top2α in de novo PIC formation, and we propose that Top2α facilitates efficient activation of Pol I transcription through its ability to cleave, passage and re-ligate dsDNA and, thereby, to alter the topology of the rDNA promoter, alleviating topological constraints to PIC assembly and stability ( Fig. 7c ). At the rDNA promoter, the local topology or higher-order structure [46] , [47] of the DNA can influence transcription of the rRNA gene and can be affected by chromatin context, including binding of the architectural protein UBF, which bends and supercoils the promoter [48] , [49] , and nucleosome positioning [50] . TBP–TAF complex SL1 directs Pol I PIC formation and stabilizes UBF at the rDNA promoter [51] . We envisage that, in activation of Pol I transcription, SL1 binds to the rDNA promoter, RRN3 binds to SL1 and Top2α is recruited through its interaction with RRN3, and then Top2α-mediated cleavage, passage and re-ligation of dsDNA at the rDNA promoter creates a topological state conducive to the efficient de novo assembly and stabilization of a functional PIC, including SL1, UBF and initiation-competent Pol Iβ, so that transcription can now be initiated and re-initiated. Lack of Top2α catalytic activity during de novo PIC formation would reduce Pol I transcription activation by affecting the equilibrium of SL1 and UBF binding to the promoter and, thereby, the efficiency of Pol I recruitment. Top2α could also, potentially, facilitate efficient de novo PIC formation upon activation of rDNA transcription by stimulating promoter escape and Pol I processivity in the pioneering round of transcription. In actively growing cells, a relatively high density of Pol I complexes facilitates Pol I clustering [52] . Consequently, positive supercoils ahead of the transcribing complex and negative supercoils behind [7] , [12] could potentially be dissipated by the actions of the adjacent polymerases [52] , such that topoisomerase activity would not be required, except perhaps ahead of a stalled polymerase or in regions where the density of polymerases is sparse. A polymerase pioneering the first round of activated transcription, without the advantage of an adjacent polymerase to dissipate the supercoiling it generates as it transcribes the rDNA would require topoisomerase cleavage. In the absence of Top2α, the observed decrease in occupancy by PIC components of the rDNA promoter might be accounted for if pioneering polymerases were stalled, due to the topological constraints imposed by failure to resolve supercoiling at or before promoter escape, thereby preventing the productive interaction of incoming PIC components with the rDNA promoter. We considered the possibility that Top2α might affect serum-activated de novo PIC formation by influencing the assembly of nucleosome remodelling machineries for repositioning of nucleosomes through a mechanism similar to that proposed for DNA topoisomerase IIβ (Top2β) in ligand (hormone)-stimulated activation of Pol II promoters [19] , which involves recruitment of DNA-damage response proteins. However, such a mode of action seems unlikely, as key components of the repair machineries (such as Ku70, Ku80 and DNA-PK) were not detectable by ChIP analysis at the activated rDNA promoters (our unpublished results), suggesting that, if Top2α affects nucleosome positioning in activation of Pol I transcription, then it achieves this through alternative means. Our findings reveal a novel dimension to the efficacy of Top2 inhibitors used in cancer treatment [4] , [5] , [6] and, potentially, to the search for Top2α-specific anti-cancer agents [5] , [53] . De novo PIC formation and activation of Pol I transcription occur during each cell cycle at newly replicated rRNA genes and might also be required for the upregulation of Pol I transcription linked to cancer [26] , [27] . We have demonstrated that the Top2 inhibitor etoposide, an effective anti-cancer drug, can reduce de novo PIC assembly and activation of Pol I transcription, independently of the p53 status of cells and the ATM/ATR-dependent DNA-damage response pathways. This suggests that this Top2 inhibitor might function in part to restrict Pol I transcription by limiting de novo activation of rRNA genes, which, ultimately, could lead to the abrogation of Pol I transcription, even in p53-null cells. This would have devastating consequences for protein synthesis, constraining the runaway growth associated with cancers. Indeed, maintenance of elevated levels of Pol I activity in cancer cells appears critically important for the process of malignant transformation and cancer cell survival. For instance, CX-5461, a selective inhibitor of Pol I transcription, induced p53-dependent apoptotic cell death in the majority of Eμ-Myc lymphoma cells at concentrations that reduced Pol I transcription about 50% (ref. 54 ). Recent studies have illustrated the effectiveness of targeting Pol I transcription in anti-cancer therapy for haematological malignancies [54] and solid tumours [55] . Therefore, we speculate that inhibitors specifically designed to target Top2α in Pol I transcription (which may be less likely to cause secondary cancers than those targeting the β-isoform [53] ) could be effective non-genotoxic tools for use in the battle against cancer. Cell-culture conditions and Top2 depletion or inhibition U2OS cells in McCoy’s 5A medium plus 10% FBS, H1299 cells (homozygous partial deletion of p53) in RPMI plus 10% FBS and HTETOP cells (derivative of human fibrosarcoma cell line HT1080) in DMEM high glucose (4.5 g l −1 ) plus 10% FBS and other additives [33] were grown to ~60–70% confluency, washed twice with Dulbecco’s PBS and then serum-starved for 20 h in DMEM low glucose (1 g l −1 ). For activation of Pol I transcription, serum-starved cells were incubated in DMEM low glucose (1 g l −1 ) containing 20% FBS. For Top2 inhibition, Top2 poison etoposide (100 μM final concentration; Merck) or catalytic inhibitors ICRF-193 (50 μM) and merbarone (100 μM; Merck) were added (except Fig. 6g ). For Top2α depletion, HTETOP medium was supplemented with 1 μg ml −1 Tet for 48 h. Cell and in vitro expression of GFP-Top2α fusion proteins HTETOP cells expressing GFP-Top2α were as described (Clone H [33] ). Stop codons were introduced into pGFP-Top2α [33] by Quickchange site-directed mutagenesis (Agilent Technologies; see Supplementary Fig. S2 ). pGFP-Top2α-WT (full-length human; 1,531 amino acids) or pGFP-Top2α-st1 (stop-codon mutant) plasmids [33] ( Not I-linearized) were electroporated into HTETOP cells, puromycin-resistant colonies were selected and single GFP-positive colonies were expanded. In vitro transcription/translation experiments used pGFP-Top2α-WT and -st5. Immunocytochemistry Cells were fixed (10 min, 4% paraformaldehyde), permeabilized (10 min, 1% Triton X-100) and blocked (10 min, 1% donkey serum in PBS), and then incubated (1 h) with antibodies ( Supplementary Table S1 ) in the blocking buffer, washed X3 for 10 min in PBS and incubated (1 h) with labelled secondary antibodies ( Supplementary Table S1 ). After washes, cells were mounted with Vectashield containing 4′,6-diamidino-2-phenylindole and visualized using confocal microscopy. RNA labelling in cells and rRNA analysis Labelling of RNA in cells (~70% confluent or ~50% for starved/refed) involved 10 μCi 3 H-uridine for ~0.2–0.4 × 10 5 cells per well of a six-well plate. In pulse-chase labelling, cells were incubated for 2 h with 3 H-uridine, washed and incubated in unlabelled medium containing 0.5 mM uridine (+/− Top2 inhibitors). RNA was extracted (RNeasy Mini Kit (Qiagen)). An amount of 2 μg of 3 H-labelled total RNA was run on a 1% formaldehyde agarose gel at 130 V for 90 min in X1 MOPS, blotted onto Hybond-N membrane (Amersham), cross-linked (ultraviolet cross-linker; UVP), analysed by tritium imaging using Fuji Tritium image plate (or following PerkinElmer En3Hance spray, exposed to Kodak Biomax XAR film at −80 °C) and then quantified using Aida software. S1 nuclease protection analysis of pre-rRNA levels Total RNA isolation from cells (~70% confluent or ~50% for starved/refed) and S1 nuclease protection analysis were performed with a 5′ end-labelled oligonucleotide probe complementary to the first 40 nucleotides of the 47S pre-rRNA transcript [44] . In vitro transcription assays Non-specific transcription assays were performed as described [28] . Run-off transcription reactions were performed essentially as described [37] , using immobilized rDNA fragments containing the human rRNA gene promoter, supplemented with purified SL1 and recombinant UBF [56] . Reactions were terminated by addition of RTL buffer and RNA transcripts (purified using RNeasy mini kits (Qiagen)) were electrophoresed on denaturing 4% acrylamide/8 M urea gels, visualized by phosphorimaging FLA-7000 (Fuji) and analysed with Aida software. Decatenation assay DNA topoisomerase II activity was assayed by analysing decatenation of kinetoplast DNA (TopoGen), according to the manufacturer’s protocols. AMP-PNP was substituted for ATP (200 and 100 μM) or Top2 inhibitor etoposide (250 and 100 μM) was included in some reactions. DNA products were resolved on a 1% agarose gel in TBE buffer. Immunoblotting and immunoprecipitation Antibodies used for immunoblotting and immunoprecipitations (IPs) are listed ( Supplementary Table S1 ). IP of nuclear extracts, prepared as described [57] , from U2OS and HTETOP cells (±1 μg ml −1 Tet) transfected (FuGENE HD reagent; Roche) with Flag-CAST expression vector pcFCAST [32] used anti-Flag M2 magnetic beads (Sigma) (for Pol I IP) for 2 h at 4 °C. The beads were washed three times in TM10/0.15 M KCl (TM10 buffer: 50 mM Tris-HCl pH 7.9, 12.5 mM MgCl 2 , 1 mM EDTA, 10% glycerol, 1 mM sodium metabisulphite and 1 mM dithiothreitol). Washed precipitates were analysed by immunoblotting. IP of nuclear extracts from HTETOP GFP-Top2α cells used anti-GFP-antibody magnetic beads (for Top2α IP). Protein–protein interaction assays Far-western analysis was performed as described [28] . Pol Iα and β fractions were subjected to SDS–PAGE and transferred to an Immobilon-P (Millipore) membrane. After renaturation, the membrane was probed with FLAG-purified, 35 S-methionine-labelled hRRN3 and human Top2α antibody. Interactions of GFP-tagged Top2α-WT and Top2α-st5 with Flag-tagged human RRN3 were analysed using 35 S-labelled in vitro- translated proteins (TNT-coupled reticulocyte lysate; Promega) in in vitro binding assays. Proteins were immunoprecipitated from the labelling reactions using anti-GFP, anti-FLAG and anti-HA antibody magnetic beads. Human RRN3 was eluted from washed beads using Flag-peptides and incubated with GFP-Top2α-WT/-st5 on beads. After binding (75 mM KCl in TM10 buffer with 0.015% NP40 and 1 μg ml −1 BSA) for 30 min on ice, beads were washed (0.1 M KCl in TM10) and bound proteins were analysed by SDS–PAGE and autoradiography. ChIP assay Cells were subjected to cross-linking (1% formaldehyde, room temperature, 10 min; terminated by addition of glycine to a final concentration of 0.125 M for 5 min) and then chromatin was isolated as described [58] and sheered to ~300 bp of average-size fragments (Bioruptor; Diagenode). A single ChIP used chromatin from 2.5 × 10 5 or 1 × 10 6 cells and antibodies as in Supplementary Table S2 , incubated overnight at 4 °C, and then for 2 h with Protein A/G beads (Invitrogen) at room temperature. Beads were washed five times in 450 μl volume of RIPA ChIP buffer [59] and twice with 200 μl TE buffer with aid of the Precipitor (Abnova). DNA on washed beads [59] was eluted, and cross-link reversal was performed in one stage as described [60] . DNA was purified (IPure kit; Diagenode with Precipitor; Abnova) and analysed by qPCR (QuantiFast Multiplex PCR Mix; Qiagen) in triplicates using primer combinations and probes covering regions of rDNA repeat ( Supplementary Table S3 ) on Light Cycler 480-II (Roche). Results were expressed as percentage of input chromatin and normalized to control IgG levels. Bar graphs show the average from three independent experiments ( n =3); s.d. and statistical significance (probability values: *** P <0.001; ** P <0.01; and * P <0.05, for drug-treated versus control cells) have been calculated using one- and two-way analysis of variance on R software (open-source statistical computing and graphics software). DNA double-strand break detection assay Cells were fixed, permeabilized in situ and DNA breaks were labelled with biotin-11–dUTP and terminal TdT as described [19] . In brief, cells (15 cm dish per single experimental point) were washed with 37 °C PBS and fixed for 20 min with Streck Fixative (0.15 M 2-bromo-2-nitropropane-1,3-diol, 0.1 M diazolidinyl urea, 0.04 M zinc sulphate heptahydrate, 0.01 M sodium citrate dihydrate and 50 mM EDTA) at room temperature and permeabilized by further incubation for 15 min at room temperature in PM buffer (0.1 M Tris-HCl, pH 7.5, 50 mM EDTA and 1% Triton X-100). Cells were washed six times with 10 ml of water before one wash with 3 ml of X1 TdT buffer containing 0.005% Triton X-100. Cells were subsequently incubated in 4 ml reaction buffer (X1 TdT buffer, 0.005% Triton X-100, 45 μM biotin-11–dUTP (Fermentas) and 250 U ml −1 terminal deoxynucleotidetransferase (Promega)) for 90 min at 37 °C on rotating platform. Cells were washed twice with 10 ml ice-cold TBS (50 mM Tris-HCl pH 7.5, 150 mM NaCl) and then carefully collected with a large cell scraper, pelleted by centrifugation and lysed in 200 μl lysis buffer (50 mM Tris-HCl pH 8.0, 10 mM EDTA and 2% SDS) for 15 min at 37 °C. Chromatin was sheared using the Bioruptor (Diagenode) to 500 bp of average-size fragments, and diluted and biotinylated DNA fragments were captured with 50 μl of Streptavidin M280 magnetic beads (Invitrogen) for 2 h at room temperature. Beads were washed five times in 450 μl of RIPA ChIP buffer [59] and twice in 200 μl TE buffer with the aid of a Precipitor (Abnova). DNA elution was performed as described [60] . Purified DNA was analysed by qPCR using QuantiFast Multiplex PCR Mix (Qiagen) and the rDNA promoter-specific combination of primers and probe (see Supplementary Table S3 ) on Light Cycler 480-II (Roche). For the glyceraldehyde-3-phosphate dehydrogenase promoter control, we used the following forward and reverse primers: 5′-CAACGGATTTGGTCGTATTGG-3′ and 5′-TGATGGCAACAATATCCACTTTACC-3′ with the probe 5′-TCACCAGGGCTGCTT-3′ (Applied Biosystems). For the peptidylprolyl isomerase A gene promoter, the primers were as follows: 5′-CAAATGGTTCCCAGTTTTTCATC-3′ and 5′-TTGCCAAACACCACATGCTT-3′ with the probe 5′-CACTGCCAAGACTG-3′ (Applied Biosystems). PCR parameters were set as recommended by PCR Mix manufacturer (Qiagen). All PCR reactions were performed in triplicate and averages; s.d. and statistical significance (*** P <0.001; ** P <0.01; * P <0.05; by analysis of variance) were derived from three independent experiments ( n =3). Results were expressed as percentage of input chromatin and normalized to control reactions where no biotin-11–dUTP was added at the labelling stage. How to cite this article: Ray, S. et al. Topoisomerase IIα promotes activation of RNA polymerase I transcription by facilitating pre-initiation complex formation. Nat. Commun. 4:1598 doi: 10.1038/ncomms2599 (2013).